Oxygenated amorphous carbon for resistive memory applications Carbon-based electronics is a promising alternative to traditional silicon-based electronics as it could enable faster, smaller and cheaper transistors, interconnects and memory devices. However, the development of carbon-based memory devices has been hampered either by the complex fabrication methods of crystalline carbon allotropes or by poor performance. Here we present an oxygenated amorphous carbon (a-CO x ) produced by physical vapour deposition that has several properties in common with graphite oxide. Moreover, its simple fabrication method ensures excellent reproducibility and tuning of its properties. Memory devices based on a-CO x exhibit outstanding non-volatile resistive memory performance, such as switching times on the order of 10 ns and cycling endurance in excess of 10 4 times. A detailed investigation of the pristine, SET and RESET states indicates a switching mechanism based on the electrochemical redox reaction of carbon. These results suggest that a-CO x could play a key role in non-volatile memory technology and carbon-based electronics. The extraordinary mechanical, optical and electrical properties of graphene [1] , graphene oxide [2] and carbon nanotubes [3] have the potential to overcome the limitations of traditional complementary metal-oxide semiconductor technology, paving the way towards so-called carbon-based electronics [4] . Another fascinating development in the field of nanoelectronics is that of memristive devices or resistive memory devices. These devices are poised to play a key role in both conventional [5] and non-von Neumann computing [6] , [7] , [8] . In this context, there is a growing interest in carbon-based resistive memories [9] , [10] , which promise to be extremely fast, small as well as flexible and biocompatible. However, despite the large interest in resistive memories based on graphene [11] , [12] , [13] , graphene oxide [14] , [15] , [16] , [17] , [18] , [19] , [20] , [21] , [22] and carbon nanotubes [23] , [24] , [25] , [26] , their complex fabrication methods, which involve high process temperatures, the use of metal catalysts, ex situ synthesis or the production of toxic gases as a side-effect, hinder their large-scale development. These complex methods also limit their wafer-scale integration into existing complementary metal-oxide semiconductor technology or plastic electronics as well as reliable control of their properties [27] . Recently, attention has mainly focused on these novel crystalline carbon allotropes, whereas amorphous forms of carbon have been away from the spotlight despite their suitability for easy, room-temperature and wafer-scale fabrication [28] . Their chemical and electrical properties can easily be tuned, but their amorphous nature prevents them from achieving the outstanding properties of their crystalline counterparts. However, this does not preclude their use in resistive memory applications: the switching mechanism in resistive memories generally relies on the clustering of defects across disordered materials [29] , [30] , so there is no need to use crystalline forms of carbon. Quite in contrast, the use of amorphous materials could be even beneficial. Resistive memories based on amorphous carbon materials have been proposed by some research groups, including ours [31] , [32] , [33] , [34] , [35] . However, those generally suffered from limited performance, especially in terms of endurance. In this work, we present oxygenated amorphous carbon (a-CO x ) that can be deposited by a simple, wafer-scale and room-temperature physical vapour deposition (PVD) process. We demonstrate a high degree of control over the chemical, optical and electrical properties of a-CO x , which can be tuned by changing the oxygen content. We also show that a-CO x has significant potential as a resistive switching material by the fabrication and characterization of a-CO x -based memory devices down to 100 nm dimensions. A discussion on the possible switching mechanism is also presented. Oxygenated amorphous carbon Compared with the more widely studied graphite oxide (GO), a-CO x is easier to produce and its composition can be easily altered. As illustrated in Fig. 1 , GO is mainly produced by ex situ wet oxidation of graphite flakes [2] . Wet oxidation enables the crystal structure of graphite to be preserved and single layers of graphene oxide to be dissolved in solution. However, it does not allow the properties of GO to be tuned with good reproducibility and on a wafer scale [2] , [36] . Moreover, GO flakes are transferred onto the substrate only at a later stage of the fabrication process and with poor wafer coverage, unless sophisticated filtration methods are used [37] . In contrast, a-CO x is produced by PVD of a graphitic carbon target in oxygen. PVD is a wafer-scale, bottom-up and in situ fabrication method, which allows the properties of a-CO x to be tuned with a high degree of control. 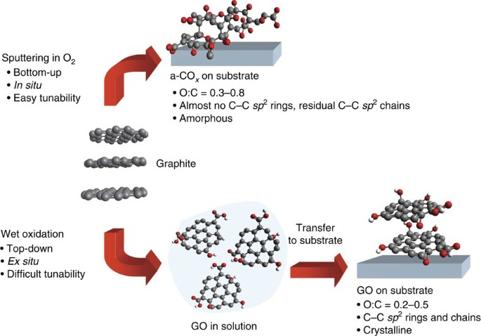Figure 1: Comparison of the fabrication methods of GO and a-COx. GO is normally produced by wet oxidation of graphite flakes, which results in widely varying and not easily tunable properties. Moreover, it is a top-down andex situapproach, as the deposition of flakes of GO onto a substrate for device fabrication, is possible only at a later stage in the process. In contrast, a-COxis produced by PVD of a graphite target in oxygen forming gas. PVD is an easy, large-scale andin situfabrication method, and amenable to tuning of the chemical and electrical properties of a-COxlayers. Figure 1: Comparison of the fabrication methods of GO and a-CO x . GO is normally produced by wet oxidation of graphite flakes, which results in widely varying and not easily tunable properties. Moreover, it is a top-down and ex situ approach, as the deposition of flakes of GO onto a substrate for device fabrication, is possible only at a later stage in the process. In contrast, a-CO x is produced by PVD of a graphite target in oxygen forming gas. PVD is an easy, large-scale and in situ fabrication method, and amenable to tuning of the chemical and electrical properties of a-CO x layers. Full size image To study its composition and to assess the influence of oxygenation and thermal annealing, a thorough investigation of a-CO x was conducted using X-ray photoelectron spectroscopy (XPS) and Raman spectroscopy. For this, 4- to 30-nm-thick a-CO x layers were deposited onto Si wafers coated with a 60-nm-thick W layer. To tune the oxygen content, the oxygen partial pressure ( ) was varied from 0 to 3.5 μbar. 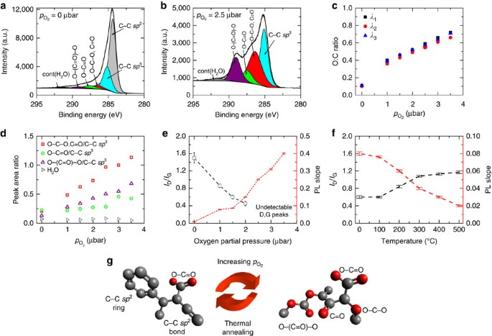Figure 2: Spectroscopic characterization of a-COx. (a,b) The comparison of XPS C1s peaks of a-C (=0 μbar) and a-COx(=2.5 μbar) indicates the absence of C–Csp2bonds and the increase of C–O groups. (c) The XPS O:C ratio, which is calculated for three different mean free path length,λ, values, and (d) the C–O groups/C–Csp3peak area ratio indicate that oxygen is increasingly being incorporated into the layers, where it bonds to carbon. (e) Visible Raman spectroscopy shows a decrease of theID/IGratio and an increase of the PL slope, confirming the reduction of C–Csp2bonds and the increase of oxygen in the layers, which saturates the non-radiative recombination centres and enables photoluminescence. There was one measurement pervalue. The error bars represent the standard deviation of the fitting error. (f) Raman spectroscopy of a-COx, after 5 min of rapid thermal annealing in vacuum at temperatures increasing from 100 to 500 °C, reveals a decrease of the PL background and an increase of theID/IGratio for increasing annealing temperatures, indicating clustering of the C–Csp2chains into rings and the release of oxygen. There was one measurement per annealing temperature. The error bars represent the standard deviation of the fitting error. (g) Evolution of the chemical bonds in a-COx: oxygen inclusion breaks the C–Csp2rings, which predominate in amorphous carbon. By increasing, the number of C–O groups increases so that a-COxmostly contains C–Csp3bonds and C–O groups with only small C–Csp2chains. Conversely, when the a-COxsamples are subjected to thermal annealing, carbon bonds rearrange into C–Csp2rings, whereas oxygen is gradually being released from the layers. Figure 2a,b compare the XPS C1s peaks of 15-nm-thick a-C ( =0 μbar) and a-CO x ( =2.5 μbar) samples, respectively. As inferred by the presence of O1s and C–O peaks in the C1s spectrum, O 2 is incorporated in a-C because of the presence of oxygen in the background pressure of the PVD chamber. With increasing , C–C sp 2 bonds are no longer detected, and a-CO x mainly consists of C–C sp 3 bonds and of C–O groups identified as epoxyl C–O, carbonyl C=O, carboxyl O–C=O and carbonate O–(C=O)–O [38] , [38] . The O:C ratio calculated from the peak area ratio O1s/C1s varies from ∼ 0.1 in a-C to ∼ 0.3 in a-CO x for =1 μbar up to ∼ 0.8 for =3.5 μbar, as shown in Fig. 2c , where three different values of the inelastic mean free path, λ , were chosen [40] , [41] , [42] for quantification. The ratio between the C1s peak areas of the different C–O groups and the peak areas of C–C sp 3 bonds increases with increasing , indicating that oxygen is increasingly being incorporated into the layers, where it is bonded to carbon ( Fig. 2d ). It is also worth noting that the XPS analysis of thinner a-CO x samples reveals that the samples are homogenous in composition over the entire thickness range, from their bulk to the interface with the bottom metal electrode. The details of the estimation of the O:C ratio and the peak fittings and bond identification are given in Supplementary Note 1 . Figure 2: Spectroscopic characterization of a-CO x . ( a , b ) The comparison of XPS C1s peaks of a-C ( =0 μbar) and a-CO x ( =2.5 μbar) indicates the absence of C–C sp 2 bonds and the increase of C–O groups. ( c ) The XPS O:C ratio, which is calculated for three different mean free path length, λ , values, and ( d ) the C–O groups/C–C sp 3 peak area ratio indicate that oxygen is increasingly being incorporated into the layers, where it bonds to carbon. ( e ) Visible Raman spectroscopy shows a decrease of the I D / I G ratio and an increase of the PL slope, confirming the reduction of C–C sp 2 bonds and the increase of oxygen in the layers, which saturates the non-radiative recombination centres and enables photoluminescence. There was one measurement per value. The error bars represent the standard deviation of the fitting error. ( f ) Raman spectroscopy of a-CO x , after 5 min of rapid thermal annealing in vacuum at temperatures increasing from 100 to 500 °C, reveals a decrease of the PL background and an increase of the I D / I G ratio for increasing annealing temperatures, indicating clustering of the C–C sp 2 chains into rings and the release of oxygen. There was one measurement per annealing temperature. The error bars represent the standard deviation of the fitting error. ( g ) Evolution of the chemical bonds in a-CO x : oxygen inclusion breaks the C–C sp 2 rings, which predominate in amorphous carbon. By increasing , the number of C–O groups increases so that a-CO x mostly contains C–C sp 3 bonds and C–O groups with only small C–C sp 2 chains. Conversely, when the a-CO x samples are subjected to thermal annealing, carbon bonds rearrange into C–C sp 2 rings, whereas oxygen is gradually being released from the layers. Full size image Visible Raman spectra of a-CO x samples consist of the D peak, due to the breathing mode of sp 2 rings, and the G peak, due to the stretching mode of sp 2 rings and chains [43] , which are superimposed on a large photoluminescence (PL) background (for more information see Supplementary Fig. 1 ). The slope of the PL background increases, whereas the I D / I G ratio decreases for increasing , see Fig. 2e . We also studied the influence of thermal annealing by subjecting the samples to 5 min of rapid thermal annealing in vacuum over a range of 100–500 °C. Raman spectroscopy shows that the PL slope decreases and the I D / I G ratio increases, see Fig. 2f . The XPS and Raman studies show that with increasing oxygen content, the number of C–C sp 2 bonds decreases, and a-CO x essentially consists of C–O groups bonded to a network of C–C sp 3 bonds, with a smaller number of C–C sp 2 chains [43] . O 2 is increasingly being incorporated into a-CO x , where it saturates the dangling bonds and enables PL, that is, radiative electron–hole recombination [44] . When a-CO x is thermally annealed, the carbon bonds reorganize themselves into C–C sp 2 rings, and O 2 is gradually released from the samples. Figure 2g schematically illustrates how the chemical bonds in the a-CO x layers change through oxidation for increasing and through reduction for increasing annealing temperatures. It is remarkable that a-CO x has several similarities to GO: It has a high electrical resistivity owing to the oxygen inclusion that breaks the C–C sp 2 (graphite-like) rings and induces C sp 3 (diamond-like) hybridization. Moreover, it is photoluminescent and graphitizes when thermally annealed. This suggests that a-CO x , like GO, could well be applied for resistive memory or in optoelectronics [45] , [46] . Here we focus on the memory application. Memory devices Resistive memory devices were fabricated by depositing an a-CO x film on a tungsten bottom electrode, which was sputtered on a Si wafer with 500 nm thick thermal SiO 2 . Either platinum, titanium or tungsten was deposited on the a-CO x layer to serve as the top electrode. The device dimensions were defined by circular cavities produced in 35-nm-thick SiO 2 layers, with diameters ranging from ≈4 μm to ≈100 nm. a-CO x was deposited into these cavities to contact the bottom electrode. This was followed by the deposition of the top electrode metal to form a sandwich structure with a-CO x in the middle. 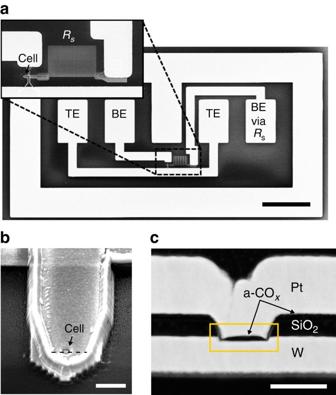Figure 3: Memory devices based on a-COx. (a) SEM top view of the top (TE), bottom (BE) and ground electrodes, which are used to electrically probe a-COxmemory cells. The series resistor is indicated withRs. Scale bar, 100 μm. (b) SEM view, under a 52° tilt angle, of the memory cell buried in the top electrode. Scale bar, 500 nm. (c) HAADF-STEM image of a typical a-COxmemory cell. The cell is circular with a diameter of 100 nm. The lamella for imaging was produced in cross section along the dashed line indicated in (b). To contact the W bottom electrode, a 18-nm-thick layer of a-COxis deposited into a cavity produced in the 35-nm-thick SiO2layer. After deposition of the Pt top electrode, a-COxis sandwiched between the two metal electrodes. Scale bar, 100 nm. Figure 3a–c show a scanning electron microscopy (SEM) top view, a zoomed-in SEM tilted (52°) view and a high-angle annular dark-field (HAADF) scanning transmission electron microscopy (STEM) cross-sectional image of a 100 nm diameter device with W as the bottom electrode and Pt as the top electrode, respectively. The intensity of the HAADF-STEM images approximately scales with the square of the atomic number and with the thickness of the sample. Thus, because of the favourable atomic number contrast, it is possible to distinguish the Pt and W layers from the SiO 2 and a-CO x layers. The device also comprises built-in series resistors ( R s ≈10 kΩ) that are used to limit the current during switching experiments. There are two paths to access the device: one with the series resistor and one without ( Fig. 3a ). Figure 3: Memory devices based on a-CO x . ( a ) SEM top view of the top (TE), bottom (BE) and ground electrodes, which are used to electrically probe a-CO x memory cells. The series resistor is indicated with R s . Scale bar, 100 μm. ( b ) SEM view, under a 52° tilt angle, of the memory cell buried in the top electrode. Scale bar, 500 nm. ( c ) HAADF-STEM image of a typical a-CO x memory cell. The cell is circular with a diameter of 100 nm. The lamella for imaging was produced in cross section along the dashed line indicated in ( b ). To contact the W bottom electrode, a 18-nm-thick layer of a-CO x is deposited into a cavity produced in the 35-nm-thick SiO 2 layer. After deposition of the Pt top electrode, a-CO x is sandwiched between the two metal electrodes. Scale bar, 100 nm. Full size image Electrical measurements Resistive switching experiments were conducted on the a-CO x -based resistive memory devices. Specifically, measurements carried out on W/a-CO x /Pt devices with 100 nm diameter are presented. a-CO x was deposited with =1.5 μbar and had a nominal thickness of 18 nm. Electrical measurements were carried out by connecting the Pt top electrode to ground and applying the signal on the W bottom electrode. The first step in the operation of the device is a forming step, see Fig. 4a . This step consists of applying a voltage pulse of positive polarity to the bottom electrode while limiting the current using the built-in series resistor. At a certain voltage value (namely, the forming voltage V form ), the current flowing through the cell abruptly increases, and the cell switches from its pristine state to a low-resistance state (LRS) also known as SET state. Note that it is possible to form a-CO x cells with relatively short pulses (for example, 1-μs-wide triangular pulses). To bring the device back to a high-resistance state (HRS) also known as RESET state, an ultra-narrow voltage pulse of negative polarity is applied to the bottom electrode without limiting the current with the R s . 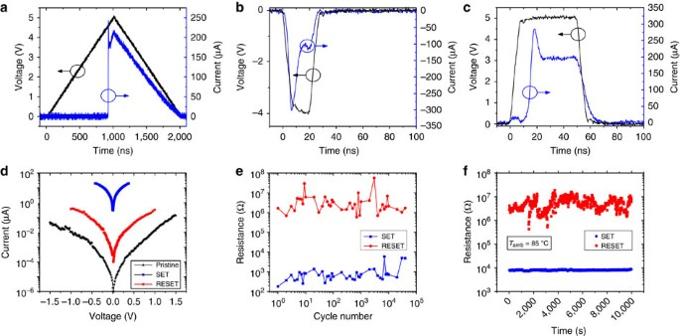Figure 4: Resistive switching in a-COx-based memory devices. (a) A typical forming pulse. At a voltage of about 5.0 V, the device switches from the pristine state to a SET state. (b) Typical RESET pulse that brings the device to a high-resistance RESET state (c) Typical SET pulse that brings the device to a SET state when applied to the RESET state. (d) Comparison of low-fieldI–Vcurves in the pristine, SET and RESET state. (e) Memory endurance tested by applying pulses of 5 V and 100 ns and −4 V and 100 ns for set and reset, respectively, and reading the resistance at 0.2 V. (f) Retention study of SET and RESET states, performed by measuring the resistance values at a voltage of 0.6 V for 104s at 85 °C. Figure 4b shows such a RESET pulse applied to the device with ≈10 ns duration and −4 V amplitude. For subsequent SET operations, pulses of positive polarity are applied to the bottom electrode with the current limiting R s in place. Figure 4c shows such a SET pulse, where a pulse with 50 ns duration and 5 V amplitude is applied to the device. The minimum pulse width decreases with increasing pulse voltage amplitude down to a limit of 50 ns for 5 V set pulses and 10 ns for −4 V reset pulses (see Supplementary Fig. 2 for more details). Figure 4: Resistive switching in a-CO x -based memory devices. ( a ) A typical forming pulse. At a voltage of about 5.0 V, the device switches from the pristine state to a SET state. ( b ) Typical RESET pulse that brings the device to a high-resistance RESET state ( c ) Typical SET pulse that brings the device to a SET state when applied to the RESET state. ( d ) Comparison of low-field I – V curves in the pristine, SET and RESET state. ( e ) Memory endurance tested by applying pulses of 5 V and 100 ns and −4 V and 100 ns for set and reset, respectively, and reading the resistance at 0.2 V. ( f ) Retention study of SET and RESET states, performed by measuring the resistance values at a voltage of 0.6 V for 10 4 s at 85 °C. Full size image The low-field I − V characteristics corresponding to a typical pristine, SET and RESET state are shown in Fig. 4d . It can be seen that both the pristine and the RESET state exhibit significant field-dependent conductivity. There is some variability in the I − V behaviour corresponding to the RESET states that is characteristic of resistive memory devices (see Supplementary Fig. 3 for more details). The endurance of the memory device was tested by applying 100 ns-long 5 V SET and −4 V RESET pulses. The resistance values read at 0.2 V after SET and RESET are presented in Fig. 4e (for clarity, only ten cycles per decade are shown). The cell could be switched for 40 k cycles with a HRS/LRS ratio of about four orders of magnitude. The test shows that a-CO x -based memory devices exhibit excellent cycling endurance compared with other carbon-based memory devices, even though our devices do not include an access transistor to control the current through the a-CO x memory cell more precisely. The stored resistance states in a-CO x cells also exhibited good retention for the entire duration of 10 4 s tested at 85 °C (see Fig. 4f ). The performance of these memory devices is significantly better than that of other carbon-based memory devices reported in the literature in particular with respect to cycling endurance which is a key challenge (see Supplementary Table 1 for a more detailed comparison). Additional studies on the electrical and resistive switching properties of a-CO x were carried out on cells having larger diameters ranging from 1 to 4 μm. 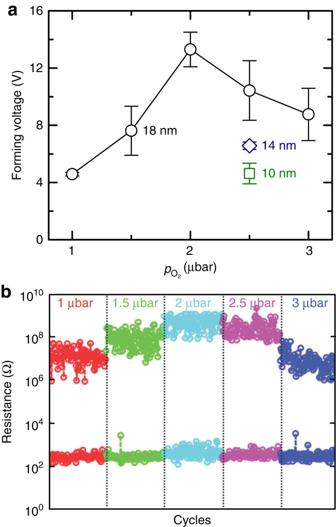Figure 5: The influence of the oxygen content. (a) Absolute values ofVformplotted as a function ofand for a-COxlayer thicknesses of 10, 14 and 18 nm. Each data point represents the average of DC measurements carried out on five different memory cells with cell diameter of 2. The error bar indicates the standard deviation.Vformincreases with increasing, reaching the saturation point at≈2 μbar. (b) RESET and SET states for increasing. The plot shows the resistance values read at 0.2 V for 100 consecutive cycles per(cell diameter of 2 μm). Although the SET state does not exhibit any significant change, the RESET state follows a trend similar to that ofVform. Figure 5a represents the values of V form as a function of . In the same plot, we also present the results of devices fabricated with thinner (14- and 10-nm-thick) a-CO x layers. Each data point is the average of measurements carried out on five different cells. V form increases with increasing oxygen partial pressure, saturating at ≈2 μbar. Figure 5b compares the SET and RESET states of a-CO x deposited at different . The plot shows the resistance values for 100 consecutive cycles per . Although the SET state does not exhibit any relevant difference, the RESET state follows a trend similar to that of V form . Figure 5: The influence of the oxygen content. ( a ) Absolute values of V form plotted as a function of and for a-CO x layer thicknesses of 10, 14 and 18 nm. Each data point represents the average of DC measurements carried out on five different memory cells with cell diameter of 2. The error bar indicates the standard deviation. V form increases with increasing , reaching the saturation point at ≈2 μbar. ( b ) RESET and SET states for increasing . The plot shows the resistance values read at 0.2 V for 100 consecutive cycles per (cell diameter of 2 μm). Although the SET state does not exhibit any significant change, the RESET state follows a trend similar to that of V form . Full size image Recently, it was shown that GO produced via Hummers oxidation of multilayer epitaxial graphene is metastable and that at room temperature its structure evolves towards a reduced form of GO [47] . As the chemical composition of a-CO x is similar to that of GO, the question arises whether a-CO x is similarly unstable. This would be an issue for resistive memory applications, as the memory retention and the reproducibility of the switching conditions over time might be compromised. Therefore, we tested the stability of a-CO x layers by checking the electrical characteristics of the same devices after six months, during which the devices were stored at ambient conditions. As shown in Supplementary Fig. 4 , we observed no major changes in the electrical resistivity of the a-CO x layers, which testifies to the good stability of this material over the time tested. Pristine, SET and RESET states A detailed investigation of the pristine, SET and RESET states was conducted to gain insight into the switching mechanism of a-CO x -based memories. In the pristine state, it is important to rule out the presence of WO x at the interface between W and a-CO x to exclude a possible interfacial switching mechanism. WO x might be present either as a native oxide or as a result of an interfacial intermixing of W and a-CO x after a-CO x deposition. The absence of native WO x was ensured during processing by depositing a-CO x right after opening the cell cavities into silicon dioxide. This procedure limits exposure of W to air and therefore limits oxidation. Moreover, as the samples were also pre-sputtered in Ar for 120 s without breaking the vacuum prior to a-CO x deposition, we ensured the removal of any native oxide up to a thickness of 5 nm. The absence of a WO x interface resulting from a possible intermixing of W and a-CO x was confirmed by energy dispersive X-ray spectroscopy (EDS) combined with electron energy-loss spectroscopy (EELS). EDS/EELS spectrum images were collected from the box marked in Fig. 3c by using a double spherical aberration-corrected STEM/TEM operated at 200 kV with a 0.4 nm pixel spacing to ensure sufficient sampling ( Fig. 6a ). The backgrounds in all EELS spectra were subtracted by fitting a decaying power-law function to an energy window just in front of the different core-loss edge onsets. 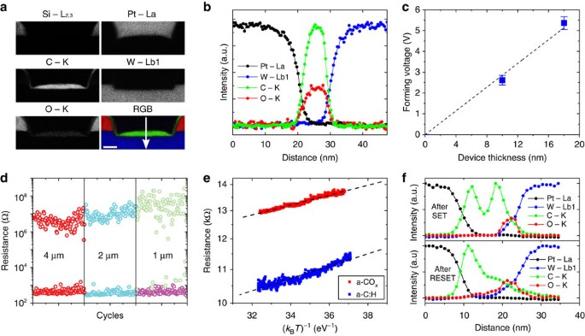Figure 6: Detailed investigation of the pristine, the SET and the RESET state. (a) Simultaneous EDS/EELS spectrum images obtained from the area outlined with a box inFig. 3cconfirm the absence of significant interfacial WOxin the pristine state. Elemental maps calculated from the EDS spectrum image (Pt–La and W–Lb1) and the EELS spectrum image (Si–L2,3, C–K and O–K). The RGB map is generated using red for O, green for C, and blue for W. Scale bar, 20 nm. (b) Intensity line-profiles laterally averaged over 50 pixels and extracted along the path indicated by a white arrow in the RGB map under (a). (c) Forming voltage as a function of device thickness, each data point is an average of measurements on five devices. The error bar indicates the standard deviation. The forming voltage scales with the thickness, confirming the bulk nature of switching as opposed to any interfacial switching mechanism. (d) Resistance values upon switching during 100 consecutive cycles for cell diameters of 4, 2 and 1 μm. The SET resistance is mostly independent of the device area and is suggestive of the SET state comprising conductive filaments. (e) Electrical transport is thermally activated for the SET states of both a-C:H and a-COxmemory devices. (f) Similarly tobthe intensity line-profiles averaged over 50 pixels were also obtained across the thickness of two different a-COxmemory cells in the SET and RESET states. They clearly show the central role played by oxygen. After forming, oxygen moves closer to the W bottom electrode leaving the a-COxlayer highly reduced. After a RESET operation, oxygen seems to move back into the a-COxlayer. Figure 6a shows the elemental maps of the Si–L 2,3 , C–K, and O–K edges extracted from the EELS spectrum image. For the EDS spectrum image, the multiple linear least squares fitting routine was used to decompose the partially overlapping Pt–La and W–Lb1 peaks. Line profiles across the entire thickness of the a-CO x memory cell were extracted from the Pt, W, C and O elemental maps ( Fig. 6b ). The results reveal a homogeneous distribution of C and O within the a-CO x memory cell, without any indication of WO x formation at the a-CO x /W interface. Note that the recess in the W electrode that is observed in the W elemental map is due to the Ar pre-sputtering aimed at removing any native oxide. High-resolution TEM images confirm the absence of significant interfacial WO x (see Supplementary Fig. 5 ). Further proof of the absence of any substantial interfacial oxide in the pristine state comes from the forming process. Figure 6c shows the forming voltage of devices with a 10 and 18-nm-thick a-CO x layer. The dependence of the forming voltage on the layer thickness confirms the bulk nature of the switching mechanism in a-CO x memories and excludes a possible interfacial switching mechanism. Figure 6: Detailed investigation of the pristine, the SET and the RESET state. ( a ) Simultaneous EDS/EELS spectrum images obtained from the area outlined with a box in Fig. 3c confirm the absence of significant interfacial WO x in the pristine state. Elemental maps calculated from the EDS spectrum image (Pt–La and W–Lb1) and the EELS spectrum image (Si–L 2,3 , C–K and O–K). The RGB map is generated using red for O, green for C, and blue for W. Scale bar, 20 nm. ( b ) Intensity line-profiles laterally averaged over 50 pixels and extracted along the path indicated by a white arrow in the RGB map under ( a ). ( c ) Forming voltage as a function of device thickness, each data point is an average of measurements on five devices. The error bar indicates the standard deviation. The forming voltage scales with the thickness, confirming the bulk nature of switching as opposed to any interfacial switching mechanism. ( d ) Resistance values upon switching during 100 consecutive cycles for cell diameters of 4, 2 and 1 μm. The SET resistance is mostly independent of the device area and is suggestive of the SET state comprising conductive filaments. ( e ) Electrical transport is thermally activated for the SET states of both a-C:H and a-CO x memory devices. ( f ) Similarly to b the intensity line-profiles averaged over 50 pixels were also obtained across the thickness of two different a-CO x memory cells in the SET and RESET states. They clearly show the central role played by oxygen. After forming, oxygen moves closer to the W bottom electrode leaving the a-CO x layer highly reduced. After a RESET operation, oxygen seems to move back into the a-CO x layer. Full size image A detailed investigation of the SET state also provides significant insight. Figure 6d shows the resistance values for 100 consecutive cycles for each cell diameter of 4, 2 and 1 μm. Despite the relatively large difference in cell diameters, the resistance in the SET state is independent of the cell area. Note that the same value of R s was used for each cell diameter. These results confirm the filamentary nature of the resistive switching in a-CO x memories, where the number and the thickness of the conductive filaments depend only on the current flowing through the cell during the SET process. To gain insight into the nature of these conductive filaments, the temperature dependence of electrical transport can be used. Figure 6e shows the temperature dependence of the SET states in an a-CO x memory device. The thermally activated transport behaviour excludes the possibility that the SET state comprises metallic filaments. This was also expected because the electrode materials are W and Pt. The most probable scenario is that the conductive filaments consist of highly reduced a-CO x , which is very similar to conductive carbon filaments. To confirm this, we produced memory cells made of the same metal electrodes, but with hydrogenated amorphous carbon (a-C:H) as switching layer. a-C:H differs from a-CO x only in the presence of C-H groups instead of C–O groups: similarly to oxygen, hydrogen reduces the number of C–C sp 2 bonds. The a-C:H devices can be formed to reach a low-resistance state as in the case of a-CO x devices (see Supplementary Fig. 6 ). Figure 6e shows the temperature dependence of the SET state in a-C:H and a-CO x resistive memories. The comparable activation energies (17.5 meV for a-C:H and 14 meV for a-CO x ) indicate that the SET state is independent of the presence of oxygen and suggest that the conductive paths of the SET state consist mainly of carbon, the common element in both a-C:H and a-CO x . During RESET, it is likely that these conductive carbon-rich filaments are partially ruptured. This could be partly due to Joule heating as in the case of memory devices based on diamond-like carbon or on a-C:H. However, in the case of a-CO x , there is also a strong chemical component to it. As we apply a positive polarity to the top electrode during RESET, oxygen ions that got trapped in the bottom electrode could get released. We believe that these oxygen ions help the RESET process substantially by chemically assisting the rupture of the conductive filaments. This process resembles the reversible oxidation demonstrated in carbon nanotubes [48] and graphene [49] . To further study this, we produced a-CO x memory devices with different metal electrodes: W/a-CO x /Pt, W/a-CO x /W and W/a-CO x /Ti. All these devices exhibited switching behaviour; however, there were notable differences. The symmetric cell W/a-CO x /W did not show any preferential polarity for the SET or the RESET operation. In contrast, in asymmetric cells, the two metal electrodes exhibit a preferential bipolar switching mode. As conventionally the voltage signal is applied on the bottom electrode of the memory cell, the best performance in a W/a-CO x /Pt cell is achieved by setting it with a voltage of positive polarity and resetting it with a voltage of negative polarity, whereas the best performance in a W/a-CO x /Ti cell is achieved by setting it with a voltage of negative polarity and resetting it with a voltage of positive polarity. This is strongly suggestive of the key role played by oxygen in the switching mechanism. Given the filamentary nature of resistance switching, isolation and direct visualization of the conductive filaments (of graphitic nature) within the bulky a-CO x cell are very challenging using microscopy techniques. However, elemental line profiles from the Pt, W, C and O elemental maps across the thickness of two different a-CO x memory cells in the SET and RESET states (see Fig. 6f ) provide strong evidence of the proposed switching mechanism. The cells comprise W bottom electrodes and Pt top electrodes. After forming, in the SET state, we observe a much higher concentration of oxygen closer to the W bottom electrode, leaving the a-CO x layer highly reduced. After a RESET operation, oxygen seems to move back into the a-CO x layer. All these results are suggestive of a switching mechanism that is based on the electrochemical redox reaction of carbon. In the pristine state, electrical transport is dominated by the bulk a-CO x that is in a high-resistance state. There is also a strong field dependence of the resistivity and, at a sufficiently high voltage, a dielectric breakdown or threshold-switching behaviour occurs: a significant current flows through the device, and the device goes into a low-resistance SET state. In this state, electrical transport is dominated by conductive filaments predominantly consisting of highly reduced a-CO x , which is similar to graphitic clusters of sp 2 -hybridized carbon atoms. A RESET state of higher resistance is recovered by application of the RESET pulse. A partial rupture of the conductive filaments occurs that is strongly assisted by the release of oxygen ions trapped in the bottom electrode. A schematic illustration of the proposed switching mechanism is shown in Fig. 7 . 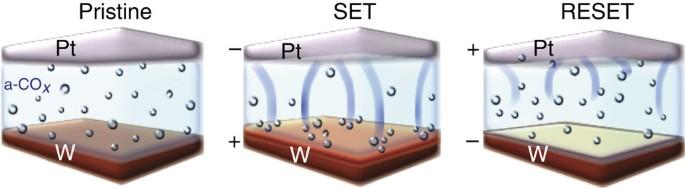Figure 7: Possible resistance switching mechanism in a-COxmemories. In the pristine state, electrical transport is dominated by the bulk a-COx. After forming, the device goes into a low-resistance SET state, in which the electrical transport is dominated by conductive filaments mostly comprised of highly reduced a-COx. Upon application of the RESET pulse, a higher-resistance RESET state is recovered by partial rupture of the conductive filaments assisted by the release of oxygen ions trapped in the bottom electrode. Figure 7: Possible resistance switching mechanism in a-CO x memories. In the pristine state, electrical transport is dominated by the bulk a-CO x . After forming, the device goes into a low-resistance SET state, in which the electrical transport is dominated by conductive filaments mostly comprised of highly reduced a-CO x . Upon application of the RESET pulse, a higher-resistance RESET state is recovered by partial rupture of the conductive filaments assisted by the release of oxygen ions trapped in the bottom electrode. Full size image When comparing a-CO x memory cells with different metal electrodes, we also observed a remarkable result. Cells with W bottom electrodes, but with different top electrodes (Pt, W and Ti) were formed by applying the same pulse of positive polarity. Interestingly, the reset current varies for the different top electrodes and increases with decreasing electron affinity of the corresponding metal (see Supplementary Fig. 7 ). The electron affinity values corresponding to Pt, W and Ti are 2.12, 0.82 and 0.085 eV, respectively, compared with 1.26 eV for C and 1.46 eV for O. In a heterogeneous material like a-CO x , the presence of various chemical bonds and configurations (with the possible presence of oligomers of C–O forming cyclic structures) may render a detailed explanation of our observation more difficult. Moreover, the exact reaction process at the interface between the a-CO x layer and the metal electrode can be rather complex as it depends on the specific nature of the interface and the type of contact (Ohmic or possible Schottky barrier and so on). However, the trend in the RESET current for the three top electrodes Pt, W and Ti can be roughly explained by the fact that carbon has a relatively high electron affinity, so that it does not oxidize easily. To make its reduction reversible, it is important to use two different electrode metals to store and release oxygen: one having a similar electron affinity to carbon such as W, and another one with a much higher value such as Pt, as an inert metal. These are indeed the electrodes that have shown the best performance in our a-CO x memory cells. Similarly, other resistive memories based on oxides, such as titanium oxide or tantalum oxide, exhibit good performance when metals such as Pt or W are used as inert electrodes, because those metals have a much higher electron affinity than Ti or Ta. In those cases Ti or Ta electrodes can serve as oxygen reservoir for the switching medium. The differences in electron affinity can also be seen in the SET states achieved after the forming process in the various devices: There is a nice correlation of the SET state resistance with the different metals used as top electrodes (see Supplementary Fig. 8 for more details). It is worth pointing out that the cycling endurance of a-CO x memory cells is much worse with W and Ti top electrodes compared with Pt electrode. The inertness of Pt electrode ensures that it does not oxidize during the RESET process when the current density is significantly higher. a-CO x memories can also be operated in a unipolar manner. This is not surprising as the RESET can also be facilitated by Joule-heating-induced rupture of the conductive filaments as in the case of carbon-based memories or a-C:H memories. However, we find that the endurance of a-CO x memories dramatically improves in the bipolar mode of operation. In summary, we have produced oxygenated amorphous carbon by PVD, an easy, room-temperature and wafer-scale deposition technique. This ease of fabrication made it possible to fine tune the chemical and electrical properties with excellent reproducibility. With increasing oxygen content, the number of C–C sp 2 bonds decreases continuously, so that a-CO x consists essentially of C–O groups bonded to a network of C–C sp 3 bonds. Consequently, a-CO x becomes increasingly photoluminescent and electrically resistive. The addition of oxygen to the amorphous carbon layer has two important benefits: (1) it induces an sp 3 hybridization of carbon, thus providing an effective and simple method for producing high-resistance amorphous carbon layers; and (2) it assists the reset of the memory cell, which now has an electrochemical nature. a-CO x shows outstanding resistive switching performance in memory cells as small as 100 nm in diameter: a switching time of 10 ns, an endurance of more than 10 4 cycles, and a tested retention of more than 10 4 s at 85 °C. Its resistive switching capability along with the ease of reproducibility and the versatility of its fabrication method make a-CO x a promising candidate for non-volatile memory applications and carbon-based electronics. Deposition of a-CO x a-CO x was deposited by DC magnetron physical vapour deposition (Von Ardenne Dresden, cluster tool CS320S) at room temperature. The PVD process was carried out with a graphitic carbon target and an O 2 +Ar mixture. DC plasma power, total pressure and total flow rate of the gas mixture were fixed at 600 W, 10 μbar and 20 sccm, respectively. To tune the O 2 content, the O 2 volumetric flow rate was varied from 0 to 35% of the volumetric flow rate of the mixture. The corresponding O 2 partial pressure ( ) varied from 0 (amorphous carbon) to 3.5 μbar, for a total pressure of 10 μbar. The PVD time was adjusted accordingly so that always about the same thickness was deposited for different values of . Before a-CO x deposition, the substrates with the bottom metal electrode (normally W) were pre-sputtered in Ar to remove any native oxide. For XPS and Raman spectroscopy analysis, 4–30-nm-thick layers of a-CO x were deposited with different on Si wafers consisting of a 500-nm-thick, thermally grown SiO 2 layer and a 60-nm-thick sputtered W layer on a 10-nm-thick Ti adhesion layer. For thermal annealing experiments, the a-CO x layers were subjected to 5 min of rapid thermal annealing in vacuum (1 × 10 −5 mbar) at temperatures increasing from 100 to 500 °C. Device fabrication The memory devices were fabricated on Si wafers with 500-nm-thick thermally grown SiO 2 . The bottom electrodes were made of 60-nm-thick sputtered metal (tungsten), which was deposited on 10-nm-thick Ti adhesion layers. Next, a 35-nm-thick layer of SiO 2 was sputtered on top of the bottom electrodes, and cavities of 35nm depth and 100 nm to 4 μm diameter were defined by electron-beam and optical lithography and etched by reactive ion etching. Then, a-CO x layers of varying thicknesses were deposited to fill the cavities. Finally, a 100-nm-thick Pt, W or Ti layer was deposited by thermal evaporation as top electrode. Microscopy and sample preparation SEM and STEM analysis, including cross sectioning and lamella preparation, were carried out by means of a FEI Helios Nanolab 450S focused ion beam (FIB) operated at accelerating voltages of 10 and 30 kV for SEM and STEM, respectively. TEM and STEM-EDS/EELS measurements were performed using a double spherical aberration-corrected JEOL JEM-ARM200F microscope operated at 200 kV, and equipped with a JEOL Dry SD100GV silicon drift detector with 100 mm 2 detection area for EDS analysis, and a Gatan Enfinium EELS spectrometer. To cover a large energy range in EELS, the dispersion was set to 0.5 eV per channel. The energy windows used to form the EELS images were 50, 100 and 100 eV for the Si–L 2,3 , C–K, and O–K edges, respectively. The annular semi-detection range of the annular dark-field detector was set to collect electrons scattered between 90 and 370 mrad. Finally, the dimensions of the EDS/EELS spectrum images shown in Fig. 6a are 300 × 120 pixels, with 0.4 nm pixel spacing and a dwell of 0.1 s per pixel. Material characterization XPS measurements were performed using a monochromatic Al K α X-ray source ( λ =1,486.74 eV) and a Phoibos 150 hemispherical analyser. The photo-emitted electron detection angle θ , defined with respect to the sample normal, was 50°, whereas the radiation-source to detector angle γ was 68.3°. The zero of the energy axis was calibrated on clean silver and gold reference samples, with Ag 3 d 5/2 at 368.27 eV, Au 4 f 7/2 at 84.00 eV, and the Fermi edge of the metals at 0 eV. The transmission function of the system, T ( E ), was determined on clean Au and Ag samples. Raman spectroscopy was carried out using a HeNe laser ( λ =632.8 nm, power <400 μW) in a single-stage confocal Raman spectrometer (Horiba Scientific LabRam HR). In all experiments, the laser was focused onto the sample surface by a × 100 objective, and the spectra were collected with a 300 lines per mm grating, averaging three spectra acquired over 30 s. The I D / I G ratio was estimated by fitting the Raman spectra with Lorentzian functions. The values of the PL backgrounds were estimated from the slope of the fitted linear background. Electrical characterization A Keithley 2400 SMU was used for DC voltage or current outputs and the measurement of the corresponding current or voltage at the sample. An Agilent 81150A Pulse Function Arbitrary Generator was used for AC voltage outputs (cell switching) and a Tektronix TDS3054B oscilloscope for AC voltage and current measurements. Mechanical relays were used to switch between AC and DC measurements. The cell resistance was measured at a constant read voltage of 0.2 V and the current–voltage ( I – V ) characteristics were measured using the current output mode of the SMU from 1 nA to 1 mA. For the temperature dependence measurements, the devices were mounted on an invar block with two embedded tungsten heaters. The temperature was measured using a thermocouple inserted into the invar block and controlled via a Eurotherm temperature controller. How to cite this article: Santini, C. A. et al. Oxygenated amorphous carbon for resistive memory applications. Nat. Commun. 6:8600 doi: 10.1038/ncomms9600 (2015).